Calculating metalation in cells reveals CobW acquires CoIIfor vitamin B12biosynthesis while related proteins prefer ZnII Protein metal-occupancy (metalation) in vivo has been elusive. To address this challenge, the available free energies of metals have recently been determined from the responses of metal sensors. Here, we use these free energy values to develop a metalation-calculator which accounts for inter-metal competition and changing metal-availabilities inside cells. We use the calculator to understand the function and mechanism of GTPase CobW, a predicted Co II -chaperone for vitamin B 12 . Upon binding nucleotide (GTP) and Mg II , CobW assembles a high-affinity site that can obtain Co II or Zn II from the intracellular milieu. In idealised cells with sensors at the mid-points of their responses, competition within the cytosol enables Co II to outcompete Zn II for binding CobW. Thus, Co II is the cognate metal. However, after growth in different [Co II ], Co II -occupancy ranges from 10 to 97% which matches CobW-dependent B 12 synthesis. The calculator also reveals that related GTPases with comparable Zn II affinities to CobW, preferentially acquire Zn II due to their relatively weaker Co II affinities. The calculator is made available here for use with other proteins. Paradoxically, in vitro, most metalloproteins prefer to bind incorrect metals [1] , [2] . A non-cognate metal may bind more tightly to the native site or bind by using a subset of the native ligands, by recruiting additional ligand(s) and/or by distorting the geometry of a binding site. Some enzymes are cambialistic and can function with alternative metals [3] , but more commonly a non-cognate metal inactivates an enzyme [4] , [5] . Correct metalation occurs in vivo because cells control the availability of metals to nascent proteins [1] , [6] , [7] , [8] . For example, specialised delivery proteins support metal acquisition by about a third of metalloproteins, (which in turn represent about a third of all proteins and about a half of all enzymes) [1] , [8] . However, metal delivery proteins do not ultimately solve the challenge of metalation because now the correct metal must somehow partition onto the delivery protein. For metalloproteins generally, there is a need to relate metal binding to the intracellular availability of metals. Our recent work provides the basis for such contextualisation [9] . Cells are thought to assist protein metalation by maintaining availabilities to the opposite of the Irving-Williams series with weaker binding metals such as Mg II , Mn II and Fe II highly available and tighter binding metals such as Ni II , Zn II and Cu I at low availabilities [10] , [11] , [12] . We have demonstrated this to be correct by determining the sensitivities of the DNA-binding metal-sensing transcriptional regulators of Salmonella enterica serovar Typhimurium (hereafter Salmonella ) [9] . The sensors trigger expression of genes whose products, for example, import metals that are deficient or export those in excess [6] , [13] . A collection of thermodynamic parameters were measured for each sensor and used to calculate the (dynamic range of) buffered intracellular metal concentrations to which each sensor is finely tuned to switch gene expression [9] , [14] . For the more competitive metals, detection is so sensitive as to suggest that there is no hydrated metal in the cell [9] , [10] . Instead, rapid associative metal-exchange can occur between labile ligands in the crowded cytosol and the binding sites of metalloproteins, making it unhelpful to express metal availabilities as concentrations of the (largely irrelevant and negligible) hydrated species: thus, the chemical potentials of the bound available metals were expressed as free energies Δ G [9] . It is hypothesised that metal-delivery proteins acquire their metals from these exchangeable, buffered pools. By reference to available Δ G values and by assuming an idealised cell in which the sensors are at the mid-points of their dynamic ranges, the correct metal (Co II ) was previously predicted to partition to the known chelatase of the anaerobic cobalamin biosynthetic pathway, CbiK [9] . There is a need to build upon this approach to account for (1) multiple competing metals and (2) non-idealised (conditional) cell cultures in order to understand the actions of putative metal delivery proteins (such as CobW and related GTPases) and to simplify such calculations for general use. The G3E GTPase superfamily contains two branches of delivery proteins involved in the assembly of Ni II centres (HypB, UreG), one for handling the cobalamin cofactor (MeaB), plus a fourth family, COG0523, investigated here [15] , [16] . Though ubiquitous, from bacteria to plants and humans, members of COG0523 have been persistently enigmatic [16] . Gene context and informatics have linked subgroups of the COG0523 family to at least three different metals: these include Nha3 associated with Fe III -requiring nitrile hydratases [17] , [18] , [19] , various subgroups (including YeiR, ZigA and ZagA) implicated in Zn II metallostasis [16] , [20] , [21] , [22] , [23] , [24] , and CobW associated with the aerobic biosynthesis of cobalamin (vitamin B 12 ) and hence Co II (ref. [25] ). Metal insertion into the preformed corrin ring in the aerobic pathway for vitamin B 12 biosynthesis appears to be irreversible [26] , [27] , highlighting the importance of Co II specificity at this step. Disruption of cobW impairs B 12 biosynthesis [25] , and a role in Co II delivery has been suggested [28] , but not established. The roles of YeiR and YjiA (two homologues of CobW in Salmonella ) are undefined, albeit Zn II has been predicted for YeiR [16] , [20] , and Co II , Ni II and Zn II shown to bind Escherichia coli (E. coli) YjiA in vitro [21] . The impact of GTP binding on metal binding remains to be tested for COG0523 GTPases. Vitamin B 12 is an essential nutrient for human health but is neither made nor required by plants [29] . Prokaryotes present in the ruminant microbiome produce B 12 and hence meat and dairy products provide a dietary source [30] . Vitamin B 12 supplements are recommended for those on a vegan diet and its biomanufacture is in demand [31] . E. coli has significant advantages over currently employed production strains [32] . Native E. coli does not make vitamin B 12 but strains containing functional B 12 pathways have been created: the most promising of these use genes of the aerobic pathway, primarily from Rhodobacter capsulatus , and produce high levels of metal-free corrinoids [33] , [34] , [35] . In R. capsulatus , Co II is inserted into the corrin ring by a cobalt chelatase ATPase (CobNST) [36] , putatively via CobW [28] . An understanding of Co II -availability inside engineered E. coli strains (referred to hereafter as E. coli* ) is required to optimise Co II supply for the B 12 pathway, with relevance to biomanufacturing. High B 12 production coupled with similarity between the metal sensors of E. coli and Salmonella also make this system tractable for testing metalation in vivo: the metal sensors of Salmonella having been thermodynamically characterised [9] . Here we calculate intracellular metalation to discover which metals partition onto three proposed metal delivery proteins (CobW, YeiR and YjiA). This work makes it widely possible to quantify metal occupancy of proteins and other molecules in vivo based on thermodynamic parameters. The cognate metals of proteins can thus be identified where this was uncertain, and the contributions of additional mechanisms that enable metalation (such as molecular interactions or bespoke growth conditions) exposed. We determine metal affinities of CobW, YeiR and YjiA, and calculate their in vivo metal occupancies (in Salmonella and closely related species), establishing that CobW cannot acquire Co II from the intracellular milieu in the absence of Mg II GTP and revealing Zn II as the preferred metal for Mg II GTP-YeiR and Mg II GTP-YjiA. Predictions of Co II occupancy of Mg II GTP-CobW in Co II -supplemented media are reflected in CobW-dependent production of B 12 in E. coli *, establishing the function of CobW in Co II -supply for B 12 and further validating an easy-to-use metalation calculator. Guanine nucleotides create two metal sites in CobW The first objective was to measure the Co II affinities of the form of CobW that acquires metal inside a cell. A modelled structure of CobW (Fig. 1a ) showed hypothetical nucleotide-binding sequences adjacent to a putative metal-binding motif, CxCC, and both of these features are conserved in the COG0523 subfamily [15] , [16] . To assess the effect of nucleotides on metal binding, CobW was overexpressed and purified (Fig. 1b and Supplementary Fig. 1 ). The protein mass determined by electrospray ionisation mass spectrometry (ESI-MS) (37,071 Da; Fig. 1c ) is consistent with that expected for CobW after cleavage of the N-terminal methionine (37,072.6 Da). Fig. 1: Co II binding to CobW is enhanced by guanine nucleotides. a Homology model of CobW (generated with SWISS-MODEL [67] using E. coli YjiA PDB entry 1NIJ [68] as template; image generated using CCP4 Molecular Graphics software) showing sulfur atoms from conserved CxCC motif (in yellow) and nucleotide-binding (GxxGxGKT, hhhExxG, SKxD*) motifs [15] , [16] (in red). *Ordinarily NKxD but [ST]KxD observed in some COG0523 proteins [15] . b Purified CobW analysed by SDS-PAGE (full image in Supplementary Fig. 1 ; n = 1 under these conditions). c ESI-MS analysis (de-convoluted spectra) of purified CobW. d Representative ( n = 2) apo-subtracted spectra of Co II -titrated CobW (26.1 µM); feature at 315 nm (inset) shows a non-linear increase. e Representative ( n = 2) elution profile following gel-filtration of a mixture of CobW (10 µM) and Co II (30 µM) showing no co-migration of metal (red) with protein (black). Fractions were analysed for protein by Bradford assay and for metal by ICP-MS. f Structures of nucleotides used in this work (generated using ChemDraw software). g As in d for a mixture of CobW (24 µM) and GMPPNP (60 µM); feature at 339 nm (inset) showing a linear increase saturating at 2:1 ratio Co II :CobW ( n = 2). h As in e for a mixture of CobW (10 µM), Co II (30 µM) and GMPPNP (30 µM) showing co-migration of 1.8 equivalents Co II per CobW (mean value from peak integration, n = 2 independent experiments). Data replicates are shown in Supplementary Fig. 1 . Full size image Co II -titration of CobW alone (26.1 µM) produced a non-linear increase in absorbance at 315 nm (Fig. 1d ) but gel-filtration of a mixture of CobW (10 µM) and Co II (30 µM) resulted in their complete separation (Fig. 1e ). Taken together, these results suggest only weak interactions between Co II and CobW in the absence of cofactors. In the presence of excess GMPPNP (60 µM), a less readily hydrolysed analogue of GTP (Fig. 1f ), Co II -titration of CobW (24 µM) produced an absorbance feature at 339 nm characteristic of ligand-to-metal charge transfer with an extinction coefficient ( ε ~2800 M −1 cm −1 ) indicative of coordination by three cysteine side-chains [37] (Fig. 1g ). Visible absorbance features (500–700 nm, ε ~300–700 M −1 cm −1 ) are characteristic of d–d transitions, diagnostic of tetrahedral Co II -coordination geometry (Fig. 1g and Supplementary Fig. 2 ). Equivalent experiments performed with GTP and an alternate stable analogue, GTPγS, generated indistinguishable spectra (Supplementary Fig. 3a, b ). These absorbance features increased linearly, saturating at 2:1 ratio Co II :CobW, and gel filtration of a mixture of CobW (10 µM) and Co II (30 µM) pre-incubated with GMPPNP (30 µM) resulted in co-migration of ~2 equivalents Co II per protein monomer (Fig. 1h ). These data show that binding of guanine nucleotides to CobW promotes tight coordination of two metal ions. Cellular [Mg II ] generates one Co II site in nucleotide-bound CobW The uniform absorbance increase observed across both metal-binding events in Fig. 1g could be explained by either the presence of two sequentially filled sites with identical spectroscopic features or two spectrally distinct sites being filled in a pairwise manner. Competition between GMPPNP-CobW and ethylene glycol tetraacetic acid (EGTA) or nitrilotriacetic acid (NTA) for Co II produced sigmoidal binding isotherms indicating positive cooperativity ( K D2 < K D1 ) between the two metal sites (Fig. 2a and Supplementary Fig. 3c, d ). Such cooperativity will result in pairwise filling of the two metal sites. Given that GTPases typically bind nucleotides in complex with Mg II , we hypothesised that the cognate metal for the first (weak-affinity) site is Mg II , and that Mg II binding triggers assembly of the second (tight-affinity) metal site in GMPPNP-CobW. Co II titration of CobW (20 µM) with GMPPNP (60 µM) and Mg II (2.7 mM, i.e. available idealised intracellular concentration, [Mg II ] cell [9] , [12] ) produced identical spectra to that observed without Mg II but saturating at 1:1 ratio Co II :CobW (Fig. 2b and Supplementary Fig. 3e ). Equivalent experiments performed with GTP and GTPγS also revealed 1:1 Co II :CobW stoichiometry in the presence of [Mg II ] cell (Supplementary Fig. 3f, g ). Thus, binding of Mg II and guanine nucleotides preassembles one distinct Co II site in CobW. Occupancy of the first site by Mg II was spectroscopically silent in these experiments. The features at 339 nm and at 500–700 nm therefore correspond exclusively to a distinct tetrahedral Co II site and the coordinating sulfhydryl side-chains likely derive (at least in part) from the CxCC motif adjacent to the nucleotide-binding site. Fig. 2: Mg II and the γ-phosphate group of GTP are necessary for high affinity Co II binding. a Absorbance (relative to Co II -free solution) of Co II -titrated CobW (20 µM) with GMPPNP (60 µM) in competition with EGTA (40 µM); titrations in the absence (black) or presence (red) of Mg II (2.7 mM, i.e. concentration in a bacterium [9] , [12] ). Data shown are representative of n = 3 independent experiments (with varying [competitor] and/or identity; see Supplementary Figs. 3c, d and 4a, b ). b Absorbance (relative to Co II -free solution) of Co II -titrated CobW (20 µM) with GMPPNP (60 µM) and Mg II (2.7 mM) in the absence of competing ligand; feature at 339 nm (inset) showing linear increase saturating at 1:1 ratio Co II :CobW ( n = 2; see Supplementary Fig. 3e ). c – e Representative K Co(II) quantification for CobW in the absence or presence of nucleotides ( n = 3 independent experiments, details in Supplementary Fig. 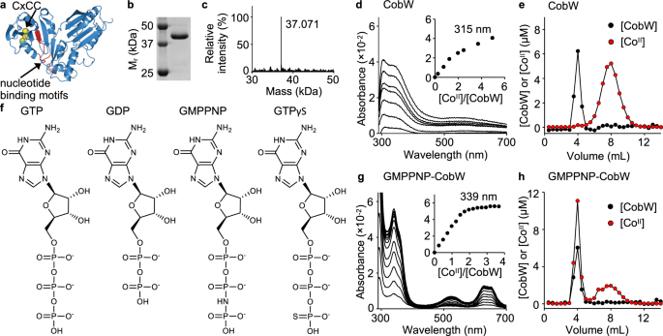Fig. 1: CoIIbinding to CobW is enhanced by guanine nucleotides. aHomology model of CobW (generated with SWISS-MODEL67usingE. coliYjiA PDB entry 1NIJ68as template; image generated using CCP4 Molecular Graphics software) showing sulfur atoms from conserved CxCC motif (in yellow) and nucleotide-binding (GxxGxGKT, hhhExxG, SKxD*) motifs15,16(in red). *Ordinarily NKxD but [ST]KxD observed in some COG0523 proteins15.bPurified CobW analysed by SDS-PAGE (full image in Supplementary Fig.1;n= 1 under these conditions).cESI-MS analysis (de-convoluted spectra) of purified CobW.dRepresentative (n= 2) apo-subtracted spectra of CoII-titrated CobW (26.1 µM); feature at 315 nm (inset) shows a non-linear increase.eRepresentative (n= 2) elution profile following gel-filtration of a mixture of CobW (10 µM) and CoII(30 µM) showing no co-migration of metal (red) with protein (black). Fractions were analysed for protein by Bradford assay and for metal by ICP-MS.fStructures of nucleotides used in this work (generated using ChemDraw software).gAs indfor a mixture of CobW (24 µM) and GMPPNP (60 µM); feature at 339 nm (inset) showing a linear increase saturating at 2:1 ratio CoII:CobW (n= 2).hAs inefor a mixture of CobW (10 µM), CoII(30 µM) and GMPPNP (30 µM) showing co-migration of 1.8 equivalents CoIIper CobW (mean value from peak integration,n= 2 independent experiments). Data replicates are shown in Supplementary Fig.1. 4 and Supplementary Table 1 ). c Fluorescence quenching of Co II -titrated fura-2 (10 µM) in competition with CobW alone (37 µM). d Fluorescence quenching of Co II -titrated fura-2 (8.1 µM) in competition with CobW (20 µM) with Mg II (2.7 mM) and GDP (200 µM). e Absorbance (relative to Co II -free solution) of Co II -titrated CobW (18 µM) in competition with EGTA (2.0 mM) with Mg II (2.7 mM) and GTP (200 µM). Solid traces in a , c , d , e show curve fits of experimental data to a model where CobW binds one molar equivalent Co II per protein monomer. Dashed lines show simulated responses for K Co(II) tenfold tighter or weaker than the fitted value. f Analysis of GTP hydrolysis by anion-exchange chromatography. Control samples of GTP and GDP elute as distinct peaks (red traces) measured by absorbance at 254 nm. Black traces show the extent of hydrolysis of GTP (200 µM) incubated with CobW (20 µM), Mg II (2.7 mM) and Co II (18 µM) over time. g Analysis of data from f showing % GTP remaining over time. After 390 min incubation, nucleotides remain primarily (>75 %) unhydrolysed. Equivalent data using 4:1 ratio GTP:CobW is shown in Supplementary Fig. 6 . Full size image Due to the tight coordination of Co II to nucleotide-bound forms of CobW (i.e. no measurable dissociation at the micromolar-range protein concentrations required for detection), it was necessary to employ competition assays, whereby Co II is partitioned between the protein and a ligand of well-matched and defined Co II affinity, for reliable quantification of metal-binding affinities [38] . Competition between Mg II GMPPNP-CobW and EGTA for Co II yielded a binding isotherm consistent with 1:1 stoichiometry for both Co II :protein and Co II :EGTA, and enabled K Co(II) of 2.7 (±0.4) × 10 −9 M for Mg II GMPPNP-CobW to be determined (Fig. 2a , Supplementary Fig. 4a, b and Supplementary Tables 1 , 2 ). Mg II had negligible impact on the conditional affinity of EGTA for Co II at the concentrations used here (Supplementary Table 3 ): For this reason, Mg II was not incorporated into curve-fitting models. 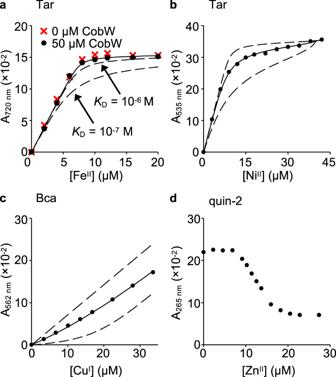Fig. 3: Binding of MgIIGTP-CobW to FeII, NiII, CuIand ZnII. aAbsorbance upon FeIItitration into a mixture of Tar (16 µM), MgII(2.7 mM) and GTP (500 µM) in the absence (red crosses) or presence (black circles) of CobW (50 µM). Dashed lines show simulated responses for specifiedKFe(II)of MgIIGTP-CobW, providing limitingKFe(II)≥ 10−6M. Control FeIItitration into a solution of Tar (16 µM) in buffer only (Supplementary Fig.8a) confirmed that MgIIand GTP did not inhibit stoichiometric FeIITar2formation.bAbsorbance change (relative to NiII-free solution) of NiII-titrated Tar (20 µM) in competition with CobW (30 µM) in the presence of MgII(2.7 mM) and GTP (300 µM).cAbsorbance of CuI-titrated Bca (1.0 mM) in competition with CobW (20 µM) in the presence of MgII(2.7 mM) and GTP (200 µM). Ina–c, solid traces show curve fits of experimental data to models where CobW binds one molar equivalent of metal per protein monomer. Supplementary Table2contains mean ± standard deviation (SD)Kmetalvalues fromn= 3 independent experiments (full details in Supplementary Figs.8–12and Supplementary Table1). Inb,c, dashed lines show simulated responses forKmetaltenfold tighter or weaker than the fitted value.dAbsorbance (relative to probe-free solution) upon titration of ZnIIinto a mixture of quin-2 (10 µM), MgII(2.7 mM), GTP (100 µM) and CobW (10 µM). Competition with EGTA revealed a Co II affinity for Mg II GTPγS-CobW ( K Co(II) = 1.7 (±0.8) × 10 −10 M; Supplementary Fig. 4c–e and Supplementary Tables 1 , 2 ), that was more than tenfold tighter than Mg II GMPPNP-CobW, establishing that the nature of the bound nucleotide exerts an effect on metal binding to CobW. Co II binds CobW 1000-fold tighter with GTP than GDP Observed variation in Co II affinities of CobW in association with Mg II GTPγS versus Mg II GMPPNP prompted us to assess the Co II affinities of all three anticipated biological species: nucleotide-free CobW, Mg II GTP-CobW and Mg II GDP-CobW. Co II affinities of CobW and Mg II GDP-CobW were determined via competition with the probe ligand fura-2 (Fig. 2c, d , Supplementary Fig. 4f–i and Supplementary Tables 1 , 2 ), which undergoes fluorescence quenching upon Co II binding [39] . Fura-2 is too weak to compete effectively with Mg II GTP-CobW (Supplementary Fig. 4j ), but high concentrations of EGTA or NTA imposed sufficient competition to enable K Co(II) of 3.0 (±0.8) × 10 −11 M to be determined (Fig. 2e , Supplementary Fig. 4k–m and Supplementary Tables 1 , 2 ). GTP concentration was not a limiting factor in these affinity measurements (Supplementary Fig. 5 ). Under identical conditions used for affinity measurements, we confirmed that CobW-catalysed GTP hydrolysis is sufficiently slow such that nucleotides remain predominantly unhydrolysed over the duration of metal-binding experiments (Fig. 2f, g and Supplementary Fig. 6 ). 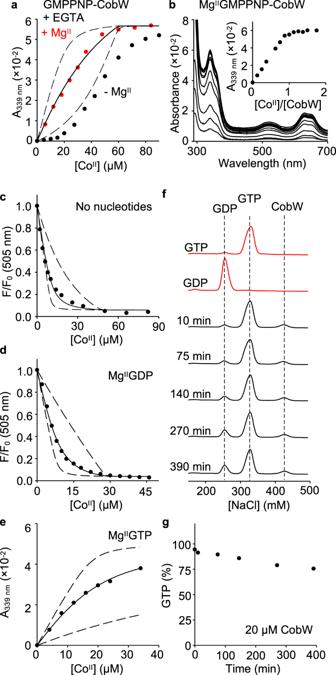Mg II GDP-CobW, despite displaying identical absorbance features indicating the persistence of the cysteine-rich tetrahedral site (Supplementary Fig. Fig. 2: MgIIand the γ-phosphate group of GTP are necessary for high affinity CoIIbinding. aAbsorbance (relative to CoII-free solution) of CoII-titrated CobW (20 µM) with GMPPNP (60 µM) in competition with EGTA (40 µM); titrations in the absence (black) or presence (red) of MgII(2.7 mM, i.e. concentration in a bacterium9,12). Data shown are representative ofn= 3 independent experiments (with varying [competitor] and/or identity; see Supplementary Figs.3c, dand4a, b).bAbsorbance (relative to CoII-free solution) of CoII-titrated CobW (20 µM) with GMPPNP (60 µM) and MgII(2.7 mM) in the absence of competing ligand; feature at 339 nm (inset) showing linear increase saturating at 1:1 ratio CoII:CobW (n= 2; see Supplementary Fig.3e).c–eRepresentativeKCo(II)quantification for CobW in the absence or presence of nucleotides (n= 3 independent experiments, details in Supplementary Fig.4and Supplementary Table1).cFluorescence quenching of CoII-titrated fura-2 (10 µM) in competition with CobW alone (37 µM).dFluorescence quenching of CoII-titrated fura-2 (8.1 µM) in competition with CobW (20 µM) with MgII(2.7 mM) and GDP (200 µM).eAbsorbance (relative to CoII-free solution) of CoII-titrated CobW (18 µM) in competition with EGTA (2.0 mM) with MgII(2.7 mM) and GTP (200 µM). Solid traces ina,c,d,eshow curve fits of experimental data to a model where CobW binds one molar equivalent CoIIper protein monomer. Dashed lines show simulated responses forKCo(II)tenfold tighter or weaker than the fitted value.fAnalysis of GTP hydrolysis by anion-exchange chromatography. Control samples of GTP and GDP elute as distinct peaks (red traces) measured by absorbance at 254 nm. Black traces show the extent of hydrolysis of GTP (200 µM) incubated with CobW (20 µM), MgII(2.7 mM) and CoII(18 µM) over time.gAnalysis of data fromfshowing % GTP remaining over time. After 390 min incubation, nucleotides remain primarily (>75 %) unhydrolysed. Equivalent data using 4:1 ratio GTP:CobW is shown in Supplementary Fig.6. 7 ), has a Co II affinity more than 1000-fold weaker than Mg II GTP-CobW and only marginally tighter than unbound CobW which lacks this site altogether (Supplementary Table 2 ). GTP also confers higher Co II affinity than either of the tested non-hydrolysable analogues in which the γ-phosphates have been modified (Fig. 1f and Supplementary Table 2 ). Thus, the presence of an intact nucleotide γ-phosphate is a prerequisite for high-affinity Co II binding. Cu I and Zn II bind Mg II GTP-CobW more tightly than Co II In view of the challenges associated with correct metal–protein speciation, we sought to determine Mg II GTP-CobW affinities for other first-row transition metals (Fe II , Ni II , Cu I , Zn II ). Fe II -titration into a mixture of Mg II GTP-CobW (50 µM) and probe ligand 4-(2-thiazolylazo)-resorcinol (Tar) (16 µM) showed Fe II being withheld by Tar which revealed a limiting affinity ( K Fe(II) > 10 −6 M) for Mg II GTP-CobW (Fig. 3a , Supplementary Fig. 8 and Supplementary Tables 1 , 2 ). Competition between Mg II GTP-CobW (10 µM) and mag-fura-2 (Mf2; 20 µM) for Ni II showed that Mg II GTP-CobW has one Ni II site which outcompetes Mf2 ( K Ni(II) < 10 −8 M) in addition to two weaker sites which compete with Mf2 for Ni II ( K Ni(II) ~10 −7 M) and are also present in CobW alone (Supplementary Fig. 9a ). Competition with Tar allowed the affinity of the tight Ni II site in Mg II GTP-CobW to be determined ( K Ni(II) = 9.8 (±6.5) × 10 −10 M; Fig. 3b , Supplementary Fig. 9b, c and Supplementary Tables 1 , 2 ). The conditional β 2 value (4.3 (±0.6) × 10 15 M −2 ) for Ni II Tar 2 formation under experimental conditions (pH 7.0, 100 mM NaCl, 400 mM KCl) was independently established by competition with EGTA (Supplementary Fig. 10 ). Titration of Mg II GTP-CobW (15 µM) and bathocuproine disulfonate (Bcs; 30 µM) with Cu I did not reach the expected intensity at saturating metal concentrations (Supplementary Fig. 11a ) suggesting the presence of a stable ternary complex, which would preclude accurate affinity determinations [40] . An equivalent experiment with alternative Cu I -probe bicinchoninic acid (Bca) showed that Mg II GTP-CobW has two Cu I sites which outcompete Bca and at least three additional weaker Cu I sites which effectively compete with the probe (Supplementary Fig. 11b ). Effective competition imposed by excess Bca enabled K Cu(I) of 2.4 (±0.9) × 10 −16 M to be determined (Fig. 3c , Supplementary Figs. 11c, d , 12 and Supplementary Tables 1 , 2 ), assuming only the tightest Cu I site can acquire metal at the limiting Cu I availabilities employed (e.g. [Cu I aq ] <3 × 10 −16 M in Fig. 3c ). Zn II titration into a mixture of quin-2 (10 µM) and Mg II GTP-CobW (10 µM) revealed one high-affinity Zn II site in the protein which was too tight to be quantified by using quin-2 thus showing K Zn(II) < 10 −12 M (Fig. 3d ). Fig. 3: Binding of Mg II GTP-CobW to Fe II , Ni II , Cu I and Zn II . a Absorbance upon Fe II titration into a mixture of Tar (16 µM), Mg II (2.7 mM) and GTP (500 µM) in the absence (red crosses) or presence (black circles) of CobW (50 µM). Dashed lines show simulated responses for specified K Fe(II) of Mg II GTP-CobW, providing limiting K Fe(II) ≥ 10 −6 M. Control Fe II titration into a solution of Tar (16 µM) in buffer only (Supplementary Fig. 8a ) confirmed that Mg II and GTP did not inhibit stoichiometric Fe II Tar 2 formation. b Absorbance change (relative to Ni II -free solution) of Ni II -titrated Tar (20 µM) in competition with CobW (30 µM) in the presence of Mg II (2.7 mM) and GTP (300 µM). c Absorbance of Cu I -titrated Bca (1.0 mM) in competition with CobW (20 µM) in the presence of Mg II (2.7 mM) and GTP (200 µM). In a – c , solid traces show curve fits of experimental data to models where CobW binds one molar equivalent of metal per protein monomer. Supplementary Table 2 contains mean ± standard deviation (SD) K metal values from n = 3 independent experiments (full details in Supplementary Figs. 8 – 12 and Supplementary Table 1 ). In b , c , dashed lines show simulated responses for K metal tenfold tighter or weaker than the fitted value. d Absorbance (relative to probe-free solution) upon titration of Zn II into a mixture of quin-2 (10 µM), Mg II (2.7 mM), GTP (100 µM) and CobW (10 µM). Full size image Because of the limiting affinity of quin-2, we employed inter-metal competition, which presumably also occurs within the buffered intracellular milieu, to determine K Zn(II) for Mg II GTP-CobW. K Zn(II) was determined, relative to the known K Co(II) , via competition between the two metals. This approach required an excess of metal ions competing for a limited number of protein metal-sites (i.e. [Co II ] tot + [Zn II ] tot > [CobW] tot ), thus it was essential to include a buffering ligand, in this case NTA, to control the speciation of all Co II and Zn II in solution (i.e. [NTA] tot > [Co II ] tot + [Zn II ] tot ). The measured equilibrium ( K ex in Fig. 4a ) was the exchange constant for Co II /Zn II exchange between the protein (Mg II GTP-CobW) and buffering ligand (NTA). Equilibrium ratios of [Co II Mg II GTP-CobW]/[Zn II Mg II GTP-CobW] were determined (Fig. 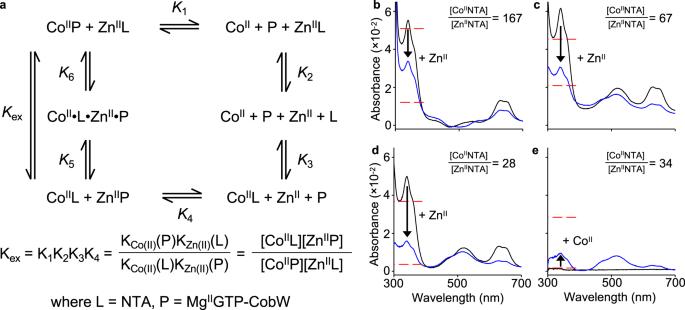Fig. 4: MgIIGTP-CobW binds ZnIIwith sub-picomolar affinity. aRepresentation of the equilibrium for exchange of CoIIand ZnIIbetween ligand (L = NTA) and protein (P = MgIIGTP-CobW).b–eAbsorbance (relative to metal-free solution) of solutions of CobW (17.9–20.4 µM), MgII(2.7 mM), GTP (200 µM) and NTA (0.4–4.0 mM) upon (b–d) first addition of CoII(black trace) then ZnII(blue trace) or (e) the reverse, at equilibrium (n= 1 for each panel). The absorbance peak at 339 nm corresponds to CoII-bound protein. An excess of ligand NTA was used to buffer both metals in each experiment: varying the ratios of ligand-bound metal ions ([CoIINTA]/[ZnIINTA] = 28–167) shifted the ratios of CoII- and ZnII-bound protein as predicted by the equilibrium exchange constant ina. ConsistentKZn(II)values for MgIIGTP-CobW were generated at all tested conditions (Supplementary Table4). Dashed red lines show expectedA339 nmpeak intensities forKZn(II)of MgIIGTP-CobW tenfold tighter or weaker than calculated values. 4b–e and Supplementary Table 4 ): absorbance intensity at A 339 nm reported specifically on the Co II –protein complex and all remaining protein was Zn II -bound (since Mg II GTP-CobW was metal-saturated under experimental conditions; Supplementary Fig. 13 ). The concentrations of NTA-bound metals were determined from mass balance relationships (Eqs. ( 6 – 8 ) in “Methods”). Experiments were conducted at multiple relative availabilities of Co II and Zn II and reciprocally (Fig. 4b–e ), with consistent results (Supplementary Table 4 ), to confirm reliability of measured affinities. We thus determined a tight K Zn(II) of 1.9 (±0.6) × 10 −13 M for Mg II GTP-CobW (Supplementary Table 2 ). Fig. 4: Mg II GTP-CobW binds Zn II with sub-picomolar affinity. a Representation of the equilibrium for exchange of Co II and Zn II between ligand (L = NTA) and protein (P = Mg II GTP-CobW). b – e Absorbance (relative to metal-free solution) of solutions of CobW (17.9–20.4 µM), Mg II (2.7 mM), GTP (200 µM) and NTA (0.4–4.0 mM) upon ( b – d ) first addition of Co II (black trace) then Zn II (blue trace) or ( e ) the reverse, at equilibrium ( n = 1 for each panel). The absorbance peak at 339 nm corresponds to Co II -bound protein. An excess of ligand NTA was used to buffer both metals in each experiment: varying the ratios of ligand-bound metal ions ([Co II NTA]/[Zn II NTA] = 28–167) shifted the ratios of Co II - and Zn II -bound protein as predicted by the equilibrium exchange constant in a . Consistent K Zn(II) values for Mg II GTP-CobW were generated at all tested conditions (Supplementary Table 4 ). Dashed red lines show expected A 339 nm peak intensities for K Zn(II) of Mg II GTP-CobW tenfold tighter or weaker than calculated values. Full size image GTP not GDP enables Co II acquisition by CobW in cells In the same manner that Fig. 3 considered competition between a ligand (Tar, Bca or quin-2) and a protein (Mg II GTP-CobW) for metal binding in vitro, metal acquisition by proteins in vivo likewise involves competition with a surplus of cytosolic ligands that buffer metals to different availabilities [8] , [9] , [14] , [41] , [42] . Recent work has estimated the buffered availabilities of metals M (where M = Mg II , Mn II , Fe II , Co II , Ni II , Cu I , Zn II ) in a reference bacterium ( Salmonella [9] ) expressed here as free energies (Δ G ; Fig. 5 ). The intracellular available Δ G for each metal, Δ G M , is defined as the free energy required for a ligand to become 50% metalated from available and exchangeable intracellular metal (see Supplementary Note 1 ). 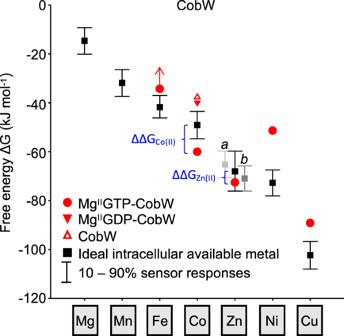Fig. 5: MgIIGTP-CobW is predicted to acquire CoIIor ZnIIin a bacterial cell. Free-energy change (ΔG) for metal binding to MgIIGTP-CobW (red circles) plotted against the intracellular available free energies for metal binding in a reference bacterial cytosol (values correspond toSalmonella) under idealised conditions (i.e. where each metal sensor undergoes half of its transcriptional response; black squares). Intracellular available ΔGZn(II)is the mean of the values determined from the two ZnIIsensors ZntR (a) and Zur (b). Bars show the change in intracellular available ΔGas cognate sensors shifts from 10–90% of their responses. Free energy differences (ΔΔG) which favour acquisition of metals by MgIIGTP-CobW in vivo are indicated in blue. ΔGvalues for CoIIcomplexes of CobW alone (open red triangle) and MgIIGDP-CobW (closed red triangle) are also shown. For FeIIbinding to MgIIGTP-CobW, arrow indicates limiting ΔG> −34.2 kJ mol−1. Figure 5 and Supplementary Fig. 14 show the intracellular available Δ G M values in an idealised cell (i.e. neither metal deficiency nor excess) defined as the metal availabilities at which the cognate sensors undergoes half of their transcriptional responses. Bars show the changes in available intracellular Δ G M as sensors shift from 10–90% (Fig. 5 ) or 1–99% (Supplementary Fig. 14 ) of their dynamic ranges. The percentage occupancy of a protein, P, with metal, M, in vivo is governed by the difference between the free energy for protein metalation, Δ G MP , and the intracellular available Δ G M (Eq. ( 1 )) and can be calculated via Eq. ( 2 ) (see Supplementary Note 1 ): 
    ΔΔG_M = ΔG_MP - ΔG_M
 (1) 
    Fractional occupancy (%) = 100 ×[ MP]/[ P]_tot = 100 ×e^ - ΔΔG_M/RT/1 + e^ - ΔΔG_M/RT
 (2) Fig. 5: Mg II GTP-CobW is predicted to acquire Co II or Zn II in a bacterial cell. Free-energy change (Δ G ) for metal binding to Mg II GTP-CobW (red circles) plotted against the intracellular available free energies for metal binding in a reference bacterial cytosol (values correspond to Salmonella ) under idealised conditions (i.e. where each metal sensor undergoes half of its transcriptional response; black squares). Intracellular available Δ G Zn(II) is the mean of the values determined from the two Zn II sensors ZntR ( a ) and Zur ( b ). Bars show the change in intracellular available Δ G as cognate sensors shifts from 10–90% of their responses. Free energy differences (ΔΔ G ) which favour acquisition of metals by Mg II GTP-CobW in vivo are indicated in blue. Δ G values for Co II complexes of CobW alone (open red triangle) and Mg II GDP-CobW (closed red triangle) are also shown. For Fe II binding to Mg II GTP-CobW, arrow indicates limiting Δ G > −34.2 kJ mol −1 . Full size image In an idealised cell, the Δ G Co(II) for CobW and Mg II GDP-CobW were both significantly more positive than intracellular available Δ G Co(II) (ΔΔ G Co(II) ≫ 0; Fig. 5 ) resulting in negligible Co II occupancies of 1.0% and 2.5% for these two protein forms, respectively. Conversely, Δ G Co(II) for Mg II GTP-CobW was significantly more negative than intracellular available Δ G Co(II) (ΔΔ G Co(II) ≪ 0), resulting in almost complete protein metalation (99%). Thus, CobW needs Mg II GTP to acquire Co II in a cell. Mg II GTP-CobW may also acquire Zn II In addition to Co II , other metals also bound to Mg II GTP-CobW (Figs. 3 and 4 ). However, ΔΔ G for Fe II , Ni II and Cu I was significantly greater than zero (Eq. ( 1 ) and Fig. 5 ), thus preventing acquisition of these metals (Eq. ( 2 ) and Table 1 ). In contrast, ΔΔ G Zn(II) was <0 with in vivo Zn II occupancy predicted to be 86% (Fig. 5 and Table 1 ). However, based on Eq. ( 2 ), the sum of metal occupancies of Mg II GTP-CobW gave an impossible total metalation >100% (Table 1 ). Since ΔΔ G was <0 for both Co II and Zn II , a more sophisticated approach needs to account for competition between multiple buffered metals in order to predict how much Zn II binds Mg II GTP-CobW in vivo. Table 1 Calculated metal occupancies of COG0523 proteins in an idealised cell a . Full size table Calculating inter-metal competition in a cell Figure 4 considered competition between Co II and Zn II for a single metal-binding site in a protein (Mg II GTP-CobW) when the metals were buffered to different availabilities in vitro by an excess of NTA. This can be represented as an available Δ G M (Supplementary Table 4 ). The observed Co II occupancy was a function of the protein’s affinities for both Co II and Zn II relative to their buffered availabilities in solution (i.e. ΔΔ G values), as described by Eq. ( 3 ) (see Supplementary Note 1 ). Fractional (%) Co^II occupancy = 100 ×e^ - ΔΔG_Co(II)/RT/1 + e^ - ΔΔG_Co(II)/RT + e^ - ΔΔG_Zn(II)/RT
 (3) By analogy, in a cytoplasm multiple metals, each buffered to different intracellular available Δ G M , compete for a single protein-binding site. We generalised Eq. ( 3 ) to account for n different metals (Eq. ( 4 ) and Supplementary Note 1 ). Fractional (% ) occupancy ( with metal M_1 of interest) = 100 ×e^ - ΔΔG_M1/RT/1 + ∑_k = 1^k = n e^ - ΔΔG_Mk/RT
 (4) Thus, we developed a metalation calculator (based on Salmonella , Supplementary Data 1 ) for determining in vivo metal occupancies of proteins, accounting for multiple inter-metal competitions plus competition from components of the intracellular milieu. Mg II GTP-CobW selects Co II in idealised ( Salmonella ) cells Since ΔΔ G was <0 for binding of both Co II and Zn II to Mg II GTP-CobW (Fig. 5 ), Eq. 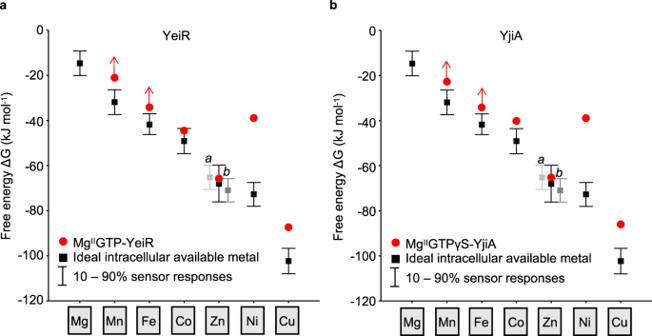Fig. 6: MgIIGTP-YeiR and MgIIGTP-YjiA preferentially acquire ZnII. aFree-energy change (ΔG) for metal binding to MgIIGTP-YeiR (red circles) plotted against the intracellular available free energies for metal binding (as described in Fig.5; black squares and bars).bAsafor MgIIGTPγS-YjiA (red circles). Arrows indicate where only a limiting ΔGwas determined (thus ΔG> plotted value). ( 4 ) was next used to predict in vivo metalation in an idealised cell. Between the five metals considered (Fe II , Co II , Ni II , Cu I and Zn II ), Mg II GTP-CobW will favour Co II binding in a cell and calculations via Eq. ( 4 ) predicted occupancies of 92% and 7%, for Co II and Zn II , respectively (Table 1 ). Thus, although Mg II GTP-CobW affinities for both Co II and Zn II are tight enough to extract either metal from the cytosolic buffer, Co II will outcompete Zn II , rationalising specificity but only in an intracellular context where there is competition from other cellular components. Related GE3 GTPase YeiR prefers Zn II in idealised Salmonella To test the calculator on a second protein, YeiR from Salmonella was overexpressed and purified (Supplementary Fig. 15 ) in order to determine metal affinities. In view of similarity between YeiR, ZigA [22] , [23] and ZagA [24] , notably a deduced binding site for Zn II -sensor Zur in the yeiR promoter (Supplementary Fig. 16 ), occupancy with Zn II might be predicted. Perhaps unexpectedly, Mg II GTP-YeiR showed a similar (slightly weaker) affinity for Zn II relative to Mg II GTP-CobW, the greatest difference in affinity was for Co II (Supplementary Figs. 17 – 21 and Supplementary Tables 5 , 6 ). Mn II failed to migrate through a gel filtration column with Mg II GTP-YeiR even when the running buffer was supplemented with an additional 20 μM MnCl 2 , revealing a Mn II affinity >2 × 10 −4 M (Supplementary Figs. 17a and 18 ). Mg II GTP-YeiR did not compete with Tar under conditions that imply Fe II affinity ≥1 × 10 −6 M (Supplementary Fig. 17b ). The Co II and Ni II affinities of Mg II GTP-YeiR were determined by competition with fura-2 and Mf2, respectively (Supplementary Fig. 17c, d and Supplementary Fig. 19a–d ). Data were fit to a 1:1 metal-binding model giving a Co II affinity of 1.5 (±0.7) × 10 −8 M and Ni II affinity of 1.5 (±0.6) × 10 −7 M. Competition for Cu I between Mg II GTP-YeiR and Bca identified a Cu I affinity of 4.9 (±5.1) × 10 −16 M (Supplementary Fig. 17e ). Competition with quin-2 was used to determine Zn II affinities of Mg II GTP-YeiR of 3.0 (±1.2) × 10 −12 M, and 4.1 (±2.7) × 10 −12 M for Mg II GTPγS-YeiR (Supplementary Figs. 17f , 19e–g , 20d and 21h, i ). Equation ( 4 ) was used to predict in vivo metalation of Mg II GTP-YeiR in an idealised cell. Zn II binding is favoured with calculated occupancies of 24% and 10%, for Zn II and Co II respectively, when sensors are at the mid-points of their dynamic ranges (Fig. 6a and Table 1 ), and trace amounts of zinc were detected after extensive purification (Supplementary Figs. 22 and 23 ). Fig. 6: Mg II GTP-YeiR and Mg II GTP-YjiA preferentially acquire Zn II . a Free-energy change (Δ G ) for metal binding to Mg II GTP-YeiR (red circles) plotted against the intracellular available free energies for metal binding (as described in Fig. 5 ; black squares and bars). b As a for Mg II GTPγS-YjiA (red circles). Arrows indicate where only a limiting Δ G was determined (thus Δ G > plotted value). Full size image Related GE3 GTPase YjiA prefers Zn II in idealised Salmonella Co II , Ni II and Zn II have all been shown to bind recombinant YjiA in vitro [21] , and the yjiA promoter contains no deduced recognition sequence for Zur. 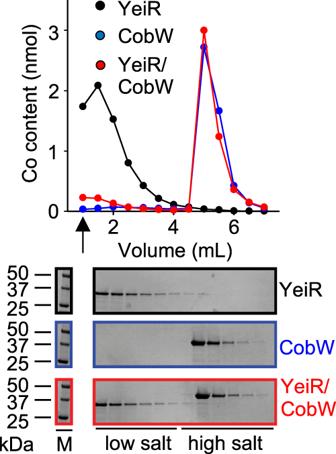Fig. 7: MgIIGTP-CobW outcompetes MgIIGTP-YeiR for CoII. Elution profile of YeiR (10 μM), CobW (10 μM) or both proteins following incubation with GTP (100 μM), MgII(2.7 mM) and CoII(8 μM) resolved by differential elution from an anion exchange column. Fractions were analysed for CoIIby ICP-MS and protein by SDS-PAGE (YeiR alone black, CobW alone blue, both proteins red;n= 1). Arrow denotes flow through fractions. Full gel images and SDS-PAGE analysis of flow through fractions shown in Supplementary Fig.26. To test the calculator on a third COG0523 protein, YjiA was overexpressed, purified (Supplementary Fig. 15 ), and its affinities for metals determined (Supplementary Figs. 24 and 25 , Supplementary Tables 5 and 7 ). Affinities were determined for Mg II GTPγS-YjiA to avoid nucleotide hydrolysis: this is supported by similar Zn II affinities being measured for Mg II GTP-YeiR and Mg II GTPγS-YeiR (Supplementary Table 5 ). Mf2 fully outcompeted Mg II GTPγS-YjiA for Mn II and simulations indicate a dissociation constant ≥1 × 10 −4 M (Supplementary Figs. 24a and 25a–c ). Mg II GTPγS-YjiA did not compete with Tar under conditions that imply Fe II affinity ≥1 × 10 −6 M (Supplementary Figs. 24b and 25d–f ). The Co II , Ni II and Cu I affinities of Mg II GTPγS-YjiA were determined using fura-2, Mf2 and Bca, respectively, as described for YeiR, giving a Co II affinity of 9.1 (±2.0) × 10 −8 M, Ni II affinity of 1.5 (±0.3) × 10 −7 M and Cu I affinity of 7.6 (±1.4) × 10 −16 M (Supplementary Figs. 24c–e and 25g–l ). Competition with quin-2 was used to determine a Zn II affinity for Mg II GTPγS-YjiA of 3.7 (±1.1) × 10 −12 M, and this was repeated with Mg II GTP-YjiA generating a near identical value of 3.3 (±2.5) × 10 −12 M (Supplementary Figs. 24f and 25m–p ). Equation ( 4 ) was used to predict in vivo metalation of Mg II GTP-YjiA in an idealised cell. Zn II binding is favoured with occupancies of 23% and 2.0% for Zn II and Co II , respectively (Fig. 6b and Table 1 ). Notably, the two Zn II sensors show a relatively wide dynamic range for Δ G Zn(II) , suggesting that Zn II occupancy could increase dependent upon media [Zn II ]. Mg II GTP-CobW outcompetes Mg II GTP-YeiR for Co II Counterintuitively, Mg II GTP-YeiR and Mg II GTP-YjiA were predicted to preferentially bind Zn II in vivo, not due to tighter affinities for Zn II , but rather due to their weaker Co II affinities relative to Mg II GTP-CobW (Table 1 , Figs. 5 and 6 , and Supplementary Tables 2 and 5 ). To test relative Co II affinities, Mg II GTP-YeiR was competed against Mg II GTP-CobW (Fig. 7 ). YeiR and CobW were incubated with Co II in the presence of Mg II and GTP, then separated by anion exchange chromatography. The chromatography was also conducted with each protein separately. Individually each protein eluted bound to Co II , but in competition Co II eluted almost exclusively with Mg II GTP-CobW (Fig. 7 and Supplementary Fig. 26 ), confirming its tighter affinity for Co II . Fig. 7: Mg II GTP-CobW outcompetes Mg II GTP-YeiR for Co II . Elution profile of YeiR (10 μM), CobW (10 μM) or both proteins following incubation with GTP (100 μM), Mg II (2.7 mM) and Co II (8 μM) resolved by differential elution from an anion exchange column. Fractions were analysed for Co II by ICP-MS and protein by SDS-PAGE (YeiR alone black, CobW alone blue, both proteins red; n = 1). Arrow denotes flow through fractions. Full gel images and SDS-PAGE analysis of flow through fractions shown in Supplementary Fig. 26 . Full size image Fine tuning ∆ G for metalation in a cell Calculated free energies for intracellular metalation (Δ G M ) in Figs. 5 and 6 are based on an assumption that cellular metal availabilities are fixed at ideal buffered concentrations where every metal sensor undergoes half of its transcriptional response (i.e. normalised fractional DNA occupancy θ D = 0.5, see ref. [9] ). In reality, cellular metal availabilities, and consequently θ D of sensors, fluctuate conditionally (e.g. in response to addition of metals or chelators to the growth media). For example, the dynamic response range (defined as θ D = 0.99–0.01) of RcnR, the Co II sensor from Salmonella , coincides with an increase in the intracellular available [Co II ] from 2.4 × 10 −11 to 2.7 × 10 −7 M, corresponding to an increase in intracellular available Δ G Co(II) from −60.6 to −37.5 kJ mol −1 (Fig. 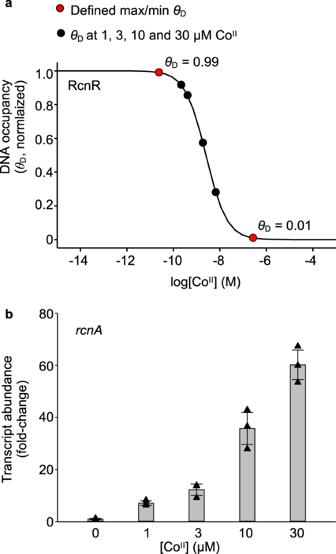Fig. 8: Calculations of conditional CoIIavailabilities in B12-producingE. coli*. aCalculated relationship between intracellular CoIIavailability and normalised DNA occupancy (θD) by RcnR.θDof 0 and 1 are the maximum and minimum calculated DNA occupancies. The dynamic range (within which RcnR responds to changing intracellular CoIIavailability) has been defined asθDof 0.01–0.99 (i.e. 1–99% of RcnR response). The calibrated maximum and minimum fold changes inrcnAtranscript abundance (i.e. boundary conditions, see Supplementary Fig.27) therefore correspond toθDof 0.01 and 0.99 in these calculations (red circles).θDfor each growth condition (black circles) was calculated from the qPCR response inb, assuming a linear relationship between change inθDand change in transcript abundance (Eq. (10)). Corresponding CoIIavailabilities are listed in Supplementary Table8.bTranscript abundance (relative to untreated control) of the RcnR-regulated genercnAfollowing 1 h exposure ofE. coli*to increasing [CoII], measured by qPCR. Data are the mean ± SD ofn= 3 biologically independent replicates. Triangle shapes represent individual experiments (some data points overlap, experimental values are available in Source Data files). 8a and Supplementary Table 8 ). Fig. 8: Calculations of conditional Co II availabilities in B 12 -producing E. coli* . a Calculated relationship between intracellular Co II availability and normalised DNA occupancy ( θ D ) by RcnR. θ D of 0 and 1 are the maximum and minimum calculated DNA occupancies. The dynamic range (within which RcnR responds to changing intracellular Co II availability) has been defined as θ D of 0.01–0.99 (i.e. 1–99% of RcnR response). The calibrated maximum and minimum fold changes in rcnA transcript abundance (i.e. boundary conditions, see Supplementary Fig. 27 ) therefore correspond to θ D of 0.01 and 0.99 in these calculations (red circles). θ D for each growth condition (black circles) was calculated from the qPCR response in b , assuming a linear relationship between change in θ D and change in transcript abundance (Eq. ( 10 )). Corresponding Co II availabilities are listed in Supplementary Table 8 . b Transcript abundance (relative to untreated control) of the RcnR-regulated gene rcnA following 1 h exposure of E. coli* to increasing [Co II ], measured by qPCR. Data are the mean ± SD of n = 3 biologically independent replicates. Triangle shapes represent individual experiments (some data points overlap, experimental values are available in Source Data files). Full size image In order to account for this variation, we developed a method to fine-tune free energy calculations under bespoke culture conditions using quantitative polymerase chain reaction (qPCR) analyses of transcripts regulated by metal sensors. Fine-tuning was performed for Co II in E. coli* which has been engineered to synthesise vitamin B 12 ( E. coli and Salmonella RcnR share 93% sequence identity and equivalent responses to available Co II were assumed). E. coli* cells were cultured in Luria-Bertani (LB) medium with increasing Co II supplementation. Abundance of the RcnR-regulated rcnA transcript (Fig. 8b ) was used to calculate θ D of RcnR for each condition (via Eq. ( 10 ) in “Methods”) following calibration of the maximum and minimum responses (defined as θ D = 0.99 and 0.01 at low and high [Co II ], respectively; Supplementary Fig. 27 ). This enabled the intracellular Co II availabilities, as conditional free energies, to be calculated from the RcnR θ D for each condition (Fig. 8a and Supplementary Table 8 ). Co II -acquisition by Mg II GTP-CobW predicts B 12 synthesis Does the amount of Co II inserted into B 12 follow the predicted metalation of Mg II GTP-CobW? Metal occupancies of Mg II GTP-CobW in E. coli* samples were recalculated (via Eq. ( 4 )) using bespoke intracellular available free energies, Δ G Co(II) , for each growth condition (Fig. 8 and Supplementary Table 8 ). This predicted that in unsupplemented LB media the protein would be predominantly Zn II -bound (10% Co II and 77% Zn II ) and that Co II occupancies would increase from 10% to 97% as added [Co II ] increased from 0 to 30 µM (Fig. 9a ). Since intracellular Zn II availability was also significant in our predictions, we confirmed that our previous estimation of Δ G Zn(II) was valid in LB media (Supplementary Fig. 28 ). Corrin concentrations (presumed to be predominantly B 12 , noting that intermediates after Co II insertion may also be detected, and that Zn II may competitively inhibit the chelatase complex but not insert into ring-contracted corrins [36] ) were measured in E. coli* strains containing or missing cobW (Fig. 9b and Supplementary Fig. 29 ), under the growth conditions for which intracellular available Δ G Co(II) was defined (Supplementary Table 8 ). As the added [Co II ] increased so did B 12 production in cobW(+) , consistent with the predicted loading of Mg II GTP-CobW with Co II (Fig. 9 ). At higher [Co II ], CobW-independent B 12 synthesis became evident. 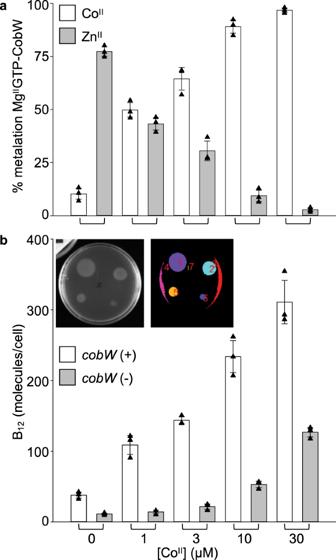Fig. 9: B12production follows predicted metalation of MgIIGTP-CobW. aPredicted metalation of MgIIGTP-CobW with CoIIand ZnII(open and grey bars, respectively) in samples treated with defined media [CoII]. Intracellular ΔGCo(II)for each condition was calculated fromrcnAexpression (Fig.8and Supplementary Table8).bB12produced byE. coli*strains with and withoutcobW(open and grey bars, respectively) following 4 h exposure to defined [CoII]. B12was detected using aSalmonellaAR2680 bioassay65(detects corrins, expected to be predominantly B12; see “Methods”) and quantified by automated analysis of growth areas (Supplementary Fig.29and Supplementary Software1). Inset shows original image and detected areas (each false coloured) for representative (n= 3) bioassay plate of B12calibration standards. All data are the mean ± SD ofn= 3 biologically independent replicates (with errors inapropagated from qPCR data in Fig.8b). Triangles represent individual experiments (some data points overlap, experimental values are available in Source Data files). As anticipated, total cellular cobalt increases with supplementation, and the amount of cobalt in B 12 is <10% of the total cellular cobalt (Supplementary Table 9 ). The number of additional atoms accumulated per cell exceeds the amount predicted if Co II were not buffered, noting that the internal buffered concentration at 10 μM exogenous Co II is 1.9 nM (Fig. 8 and Supplementary Table 8 ), and that only 1 atom per cell volume (approximately 1 femtolitre) equates to 1.7 nM. Most importantly, B 12 synthesis which is dependent on CobW (Fig. 9b , compare cobW (+) with cobW (−)) matches the trend in predicted metalation of Mg II GTP-CobW (Fig. 9a ). Fig. 9: B 12 production follows predicted metalation of Mg II GTP-CobW. a Predicted metalation of Mg II GTP-CobW with Co II and Zn II (open and grey bars, respectively) in samples treated with defined media [Co II ]. Intracellular Δ G Co(II) for each condition was calculated from rcnA expression (Fig. 8 and Supplementary Table 8 ). b B 12 produced by E. coli* strains with and without cobW (open and grey bars, respectively) following 4 h exposure to defined [Co II ]. B 12 was detected using a Salmonella AR2680 bioassay [65] (detects corrins, expected to be predominantly B 12 ; see “Methods”) and quantified by automated analysis of growth areas (Supplementary Fig. 29 and Supplementary Software 1 ). Inset shows original image and detected areas (each false coloured) for representative ( n = 3) bioassay plate of B 12 calibration standards. All data are the mean ± SD of n = 3 biologically independent replicates (with errors in a propagated from qPCR data in Fig. 8b ). Triangles represent individual experiments (some data points overlap, experimental values are available in Source Data files). Full size image Here we relate metal affinities of three putative metallochaperones to a thermodynamic framework, identifying their cognate metals which align with previous speculations [16] , [20] , [25] (Figs. 5 , 6 and Table 1 ). We establish the connection between CobW and Co II and show how CobW can acquire Co II in a cell (Figs. 1 – 5 and Table 1 ). Free-energy calculations reveal that in an idealised cell Co II ions will not flow from the cellular milieu to nucleotide-free CobW (ΔΔ G Co(II) > 0). Crucially, Co II will flow from the cellular milieu to the Mg II GTP form of CobW (ΔΔ G Co(II) < 0) (Fig. 5 , Supplementary Fig. 30a , Table 1 and Supplementary Table 2 ). Thus, CobW must first bind Mg II GTP in order to acquire Co II inside a cell. In contrast, the product of GTP hydrolysis, Mg II GDP-CobW, will release Co II to the cellular milieu (ΔΔ G Co(II) > 0) (Fig. 5 , Supplementary Fig. 30b and Supplementary Table 2 ). Thus, the GTPase activity of CobW will facilitate Co II release, for example to CobNST for insertion into the corrin ring of B 12 (Fig. 2f, g and Supplementary Fig. 6 ). We establish that CobW enhances B 12 production when Co II is limiting (Fig. 9b ), and Supplementary Fig. 30 illustrates the proposed mechanism. Zn II is identified as the preferred metal for nucleotide-bound forms of YeiR and YjiA: this is due to their weaker affinities for Co II relative to Mg II GTP-CobW (Fig. 7 and Supplementary Table 5 ), rather than tighter affinities for Zn II . These data illustrate the value of using the metalation calculator provided as Supplementary Data 1 , which can now be broadly applied to metal-speciation in the context of intracellular competition. Mg II GTP-CobW binds Zn II and Cu I more tightly than Co II (Figs. 2e , 3 , 4 and Supplementary Table 2 ), and likewise nucleotide-bound forms of YeiR and YjiA bind Cu I more tightly than Zn II . Notably, by taking into account intracellular metal availability, ΔΔ G for Cu I was shown to be greater than zero for all three proteins in idealised cells, and also in conditional cells at either 90% or 99% of the dynamic range of the Cu I sensor CueR (Figs. 5 , 6 and Supplementary Fig. 14 ). Thus, these proteins will not acquire Cu I . However, for Mg II GTP-CobW ΔΔ G for Zn II was below zero in an idealised cell suggesting mis-metalation with Zn II (Fig. 5 ). Indeed, given that CobW binds Zn II more tightly than many known Zn II proteins [14] , [43] , and comparably to YeiR and YjiA (Supplementary Tables 2 and 5 ), it seems remarkable that Zn II is not the cognate metal. The data in Fig. 4 , plus Supplementary Table 4 , illustrate how occupancies of Mg II GTP-CobW with Co II versus Zn II change as a function of relative buffered metal availabilities. By reference to intracellular available free energies, the metal with the most negative ΔΔ G will have the highest occupancy in vivo (Eq. ( 4 )). In an idealised cell, ΔΔ G for Co II is more negative than ΔΔ G for Zn II and so the weaker binding metal dominates (Fig. 5 and Supplementary Table 2 ). In contrast, for nucleotide-bound forms of YeiR and YjiA ΔΔ G for Zn II is more negative than ΔΔ G for Co II making these deduced Zn II proteins. The previously intractable challenge to understand inter-metal competition in a cell now becomes tractable. Initial calculations here, and in previous work [9] , assume an idealised cell in which the metal sensors are at the mid-points of their dynamic ranges ( θ D = 0.5). Therefore, we have calculated the available Δ G Co(II) in real (conditional) cells from the responses of RcnR ( θ D ) estimated experimentally by qPCR of rcnA (Fig. 8 and Supplementary Fig. 27 ). As with other metallochaperones [10] , [44] , CobW is crucial when the cognate metal is limiting but at elevated Co II , CobW-independent synthesis of B 12 occurs (Fig. 9b ). CobNST must acquire Co II directly from the cytosol at the higher available Δ G Co(II) . Importantly, CobW-dependent B 12 synthesis tracked with the calculated Co II occupancy of Mg II GTP-CobW in cells supplemented with different amounts of Co II (Fig. 9 ). By monitoring the responses of sensors for different metals, it will be possible to define available Δ G , and predict protein occupancies with diverse metals, in different growth conditions. The calculator should be most accurate in Salmonella and closely related species such as E. coli . However, metal availabilities can also be adjusted (and/or simulated) to account for species differences, noting that the dynamic ranges of available Δ G values might be similar even when total cellular metal changes greatly between species. Spectral features indicate that the Co II site in Mg II GTP-CobW involves thiols, likely derived from the CxCC motif in the GTPase domain, and a tetrahedral geometry (Figs. 1 , 2 and Supplementary Fig. 3 ). However, all COG0523 proteins contain the CxCC motif [16] and there is now a quest to understand why Co II affinities are weaker for Mg II GTP-bound YeiR and YjiA (and, hypothetically, ZigA and ZagA), which bind predominantly to Zn II as a result (Fig. 6 ). Notably a further pair of conserved cysteine residues (C 56 , C 61 ) in CobWs are absent from the homologues (Supplementary Fig. 31 ). Intriguingly, Ni II binding to Mg II GTP-CobW, Mg II GTP-YeiR and Mg II GTPγS-YjiA does not follow the order of stabilities of metal binding predicted by the Irving-Williams series (Figs. 5 and 6 ). An appealing explanation is that the allosteric coupling of GTP- and metal-binding imposes a (tetrahedral) geometry on the metal site that would disfavour Ni II coordination (the Irving-Williams series applies where there is no steric selection): notably, related G3E GTPases involved in Ni II homoeostasis (HypB and UreG) display square planar Ni II coordination geometry [45] , [46] . The metalation calculator has identified cognate metals for three members of the COG0523 sub-family of GE3 GTPases (Figs. 5 , 6 and Table 1 ), and this work establishes vitamin B 12 as the ultimate Co II -client of CobW (Fig. 9 ). For YeiR and YjiA, there is now a quest to identify their distinct roles and potential Zn II -requiring client(s). Under-metalation of Mg II GTP-CobW with Co II (and resultant mis-metalation with Zn II , Fig. 9a ) could be especially problematic in E. coli* due to the lack of a dedicated Co II import system in this bacterium [47] . This suggests tantalising opportunities to engineer strains suited to the manufacture of vitamin B 12 , either via enhanced Co II uptake through engineered Co II -import, or via impaired Zn II accumulation by endogenous Zn II -transport systems. By analogy, with almost a half of enzymes requiring metals, an ability to calculate metalation in vivo should have broad applicability in optimising (or subverting) metalation in biotechnology. The calculator (Supplementary Data 1 ) can be widely used to understand metalation and mismetalation of proteins that acquire Mg II , Mn II , Fe II , Co II , Ni II , Cu I or Zn II from the milieu inside living cells. Protein expression and purification The DNA sequence coding CobW was amplified by PCR using primers 1 and 2 (Supplementary Table 10 ) with genomic DNA from R. capsulatus SB1003 as template. The amplified fragment contained an NdeI restriction site at the 5ʹ end and a SpeI site at the 3ʹ end, allowing it to be cloned into a modified pET-3a vector [34] . The DNA coding sequence of yeiR (SL1344_2189) from S. enterica serovar Typhimurium strain SL1344 was obtained as a synthetic gene from Eurofins in a pEX plasmid with the T7 promoter and terminator from pET29a flanking yeiR . Additionally, the start codon of the gene (GTG) was changed to the more common ATG (pEX yeiR ). The native coding sequence of yjiA (SL1344_4461) was obtained in the same manner (pEX yjiA ). The correct sequence of each gene ( cobW , yeiR and yjiA ) was confirmed by DNA sequencing (DBS Genomics – Durham University). E. coli BL21(DE3) pLysS, transformed with either pET3a- cobW , pEX- yeiR or pEX- yjiA were cultured in LB medium with antibiotics carbenicillin (50–100 mg L −1 ) and chloramphenicol (30–34 mg L −1 ). At mid-log phase, protein expression was induced by addition of 0.4 mM (CobW), 0.5 mM (YjiA) or 1.0 mM (YeiR) IPTG. Cells were cultured (with shaking) for 3–4 h at 37 °C (CobW) or at 20 °C overnight (YeiR and YjiA). Cells were harvested and stored at −20 °C prior to use. Cells overexpressing CobW were resuspended in 20 mM sodium phosphate pH 7.4, 500 mM NaCl, 5 mM imidazole, 5 mM DTT and 1 mM PMSF for lysis (sonication) and cell debris was pelleted by centrifugation (38,000 × g , 45 min, 4 °C). Lysate was loaded to a 5-mL HisTrap HP column (GE Heathcare) pre-equilibrated in suspension buffer. CobW binds to the HisTrap column courtesy of a natural His-rich region within the protein. The column was washed with suspension buffer (10 column volumes), then eluted with suspension buffer containing 100 mM imidazole. Protein-containing fractions were incubated with excess (≥10-fold) EDTA for ≥1 h before being loaded to a HiLoad 26/600 Superdex 75 size exclusion column equilibrated in 50 mM Tris pH 8.0, 150 mM NaCl, 5 mM DTT and eluted in the same buffer. Peak CobW-containing fractions (determined from SDS-PAGE) were pooled, concentrated to ~0.5 mL (using a Vivaspin® 15 Turbo centrifugal concentrator). Protein identity was confirmed using ESI-MS by Durham University Department of Chemistry Mass Spectrometry Service. ESI-MS data were recorded on a QtoF Premier mass spectrometer coupled to an Acuity UPLC system (Waters). Protein samples were desalted prior to injection using a Waters MassPrep desalting cartridge (2.1 × 10 mm) and eluted with a linear acetonitrile gradient (20–80% v/v; 0.1% formic acid). Spectra were processed using Masslynx 4.1, deconvoluted using MaxEnt 1 and data imported into SigmaPlot software for preparation of figures. Cells overexpressing YeiR were resuspended in 20 mM sodium phosphate pH 7.4, 100 mM NaCl, 5 mM DTT, 1 mM PMSF for lysis (sonication) and cell debris was pelleted by centrifugation (31,191 × g , 15 min, 8 °C). Soluble lysate was applied to a 5-mL HisTrap column (GE Healthcare) equilibrated with lysis buffer without PMSF. The column was washed with equilibration buffer before elution with equilibration buffer containing 10, 50 and 100 mM imidazole. YeiR eluted in the buffer containing 50 mM imidazole. EDTA was added to the YeiR-containing fraction to a final concentration of 10 mM and stored overnight at 4 °C. The sample was applied to HiLoad 26/600 Superdex 75 (GE Healthcare) equilibrated with 50 mM Tris pH 8, 150 mM NaCl, 5 mM DTT and eluted with the same buffer. Peak fractions were pooled and applied to a 5-mL Q anion exchange column (GE Healthcare) equilibrated with the size exclusion column buffer. Column flow through and wash were collected before eluting the column with size exclusion column buffer with the addition of 1 M NaCl. YeiR displays no affinity for the Q column and elutes in the flow through and wash. The remaining major contaminant elutes with 1 M NaCl. The flow through and wash from the Q column were pooled and concentrated using a Spin-X UF concentrator (Corning, 10 kDa molecular weight cut-off). Cells overexpressing YjiA were resuspended in 20 mM Tris 7.5, 100 mM NaCl, 5 mM DTT, 1 mM PMSF for lysis (sonication) and cell debris was pelleted by centrifugation (two consecutive 20 min runs, 39,191 × g , 4 °C) before passing clarified supernatant through a 20-µm nylon membrane filter. Soluble lysate was applied to a 5-mL HisTrap column (GE Healthcare) equilibrated with lysis buffer without PMSF, collecting the flow through and a one column volume wash. This step removes a major contaminant which binds to the HisTrap column. Pooled flow through and wash fractions were applied to a 5-mL HiTrap Q-Sepharose fast flow column (GE Healthcare) equilibrated with lysis buffer without PMSF. The column was washed with equilibration buffer then equilibration buffer with 200 mM NaCl before elution of YjiA by application of a 50-mL gradient of 200–600 mM NaCl in equilibration buffer collecting 5 mL fractions. YjiA typically eluted between 10 and 30 mL. Fractions containing the highest concentration of YjiA with the lowest degree of contamination, as judged by SDS-PAGE, were stored overnight (4 °C) with EDTA to a final concentration of 5 mM. Fractions were concentrated to 5 mL using a Spin-X UF concentrator (Corning, 10 kDa molecular weight cut-off) and applied to HiLoad 26/600 Superdex 75 (GE Healthcare) equilibrated with lysis buffer without PMSF and eluted with the same buffer. Fractions were pooled and concentrated to 5–20 mg mL −1 using a Spin-X UF concentrator (Corning, 10 kDa molecular weight cut-off) before storage at −80 °C. Following purification, CobW, YeiR and YjiA samples were transferred to an anaerobic glovebox (Belle Technology), (0.5–1 mL) applied to a PD-10 Desalting Column prepacked with Sephadex G-25 medium (GE Healthcare) equilibrated with chelex-treated and N 2 -purged buffer (10 mM HEPES pH 7.0, 100 mM NaCl, 400 mM KCl) and eluted in the same buffer. Proteins were quantified by A 280 nm using experimentally determined extinction coefficients ( ε = 15,300 M −1 cm −1 for CobW, 52,745 M −1 cm −1 for YeiR, and 27,900 M −1 cm −1 for YjiA) determined by quantitative amino acid analysis (Alta Bioscience Ltd). Samples were confirmed to be of high purity by SDS-PAGE (full gel images are available in the Supplementary Information), and ≥92.5% (YeiR) and ≥95% (CobW, YjiA) metal-free (by inductively coupled plasma-mass spectrometry; ICP-MS). ICP-MS of one sample of YjiA was performed 3 weeks after buffer exchange and >5% zinc detected, but results were consistent with replicates containing <5% zinc. ICP-MS was conducted using Durham University Bio-ICP-MS Facility (PlasmaLab software; Thermo Fisher). Reduced thiol content was determined by reaction with ~10-fold excess of Ellman’s reagent 5,5ʹ-dithio-bis-[2-nitrobenzoic acid] (DTNB; produces one equivalent of chromophore TNB 2− per protein thiol, A 412 nm = 14,150 M −1 cm −1 ) [48] , [49] . For CobW >5.5 cysteines were found to be reactive with DTNB (expected value = 6), for YeiR 4–5 cysteines (expected value = 5), and for YjiA >4.5 cysteines (expected value = 5). Preparation of metal stocks All metal stocks were prepared in ultrapure water from appropriate salts (MgCl 2 , (NH 4 ) 2 Fe(SO 4 ) 2 , CoCl 2 , NiSO 4 , NiCl 2 , CuSO 4, ZnCl 2 , ZnSO 4 ) and quantified by ICP-MS analysis. Fe II stocks were prepared by dissolving (NH 4 ) 2 Fe(SO 4 ) 2 ·6H 2 O in deoxygenated 0.1% (v/v) HCl in an anaerobic chamber. Reaction with excess ferrozine (Fz; ∼ 50-fold) confirmed that iron was ≥95% reduced (Fe II Fz 3 ε 562 nm = 27,900 M −1 cm −1 ) [50] . Concentrated stocks were diluted daily in deoxygenated ultrapure water to prepare working solutions and confirmed to be ≥90% Fe II . Other metal stocks were prepared aerobically as concentrated stocks and diluted to working solutions with deoxygenated ultrapure water in an anaerobic chamber. Cu(I) was generated in situ (from CuSO 4 ) by hydroxylamine (1–10 mM) which quantitatively reduces Cu(II) to Cu(I) in the presence of excess chelator (L = Bca or Bcs) to form Cu I L 2 complexes [51] . Determination of CobW Co II -binding stoichiometries Metal-binding experiments were conducted in an anaerobic chamber in deoxygenated, chelex-treated 10 mM HEPES pH 7.0, 100 mM NaCl, 400 mM KCl. For stoichiometry determinations, Co II was titrated into a solution of CobW (15–30 µM) together with relevant nucleotides (supplied in ∼ 10-fold excess of protein concentration for GTP and GDP and ∼ 3-fold excess for GMPPNP and GTPγS, as specified in figure legends) in the absence or presence of Mg II (2.7 mM). Absorbance was recorded using a Lambda 35 UV-visible spectrophotometer (Perkin Elmer; UV-Win lab software). The extinction coefficient of Co II Mg II GTP-CobW ( ε 339 nm = 2800 ± 100 M −1 cm −1 , average ± s.d of n = 3 independent titrations) was determined from absorbance at saturating metal concentrations (Supplementary Fig. 3g ). Extinction coefficients of related complexes Co II Mg II GMPPNP-CobW, Co II Mg II GTPγS-CobW, Co II 2 GTP-CobW, Co II 2 GMPPNP-CobW and Co II 2 GTPγS-CobW were similarly determined (Figs. 1 , 2 and Supplementary Figs. 1 , 3 ): within experimental error, all produced the same extinction coefficient as for Co II Mg II GTP-CobW, thus ε 339 nm = 2800 M −1 cm −1 was assigned to all species. Gel-filtration chromatography experiments were performed by incubating CobW (10 µM) and Co II (30 µM) for 30 min with or without cofactor GMPPNP (30 µM) then applying 0.5 mL to a PD-10 Sephadex G-25 gel-filtration column (GE Healthcare). Eluted fractions (0.5 mL) were analysed for cobalt by ICP-MS and for protein by Bradford assay. Determination of CobW metal affinities via ligand competition Ligand competition experiments were conducted in an anaerobic chamber in deoxygenated, chelex-treated 10 mM HEPES pH 7.0, 100 mM NaCl, 400 mM KCl, except where high concentrations (≥1 mM) of competing ligand were employed, where 50 mM HEPES was used to maintain buffered pH 7.0. Absorbance was recorded using a Lambda 35 UV-visible spectrophotometer (Perkin Elmer). Fluorescence spectra were recorded using a Cary Eclipse fluorescence spectrophotometer (Agilent; Cary Eclipse scan application software). Affinities were determined at a range of different competing conditions (by varying the competing ligand and/or the protein:ligand ratio) to ensure reliability: details are documented in Supplementary Table 1 . Scripts used for data fitting (using Dynafit [52] ) are provided in Supplementary Software 2. The effect of Mg II (2.7 mM) on apparent dissociation constants of ligand standards (EGTA, NTA, fura-2, Mf2 and quin-2) was calculated to be insignificant under the conditions of competition experiments (Supplementary Table 3 ). For probes with undefined Mg II affinities (Tar, Bca), control experiments confirmed that addition of Mg II (2.7 mM) had negligible effect on competition experiments (Supplementary Figs. 10d and 12 ). Thus, Mg II was not incorporated into the curve-fitting models. For determination of weaker ( K D > 10 nM) Co II binding affinities (CobW and Mg II GDP -CobW), CoCl 2 was titrated into a solution of 5-Oxazolecarboxylic acid, 2-(6-(bis(carboxymethyl)amino)-5-(2-(2-(bis(carboxymethyl)amino)-5-methylphenoxy)ethoxy)-2-benzofuranyl)-pentapotassium salt (fura-2; quantified by ε 363 nm = 28,000 M −1 cm −1 ) [53] and CobW in the presence or absence of cofactors (MgCl 2 and GDP) and fluorescence emission ( λ ex = 360 nm; λ max ~505 nm) was recorded at equilibrium. Co II -dependent fluorescence quenching of fura-2 was used to determine Co II speciation. For determination of Co II binding affinities tighter than 10 nM (Mg II GMPPNP-CobW, Mg II GTPγS-CobW and Mg II GTP-CobW), CoCl 2 was titrated into a solution containing CobW, competing ligand (EGTA or NTA), MgCl 2 and nucleotide (GMPPNP, GTPγS or GTP). UV-visible absorbance (relative to metal-free solution) was recorded at equilibrium to determine Co II speciation ( ε 339 nm = 2800 M −1 cm −1 for Co II -bound proteins). Data were fit using Dyanfit [52] to models describing 1:1 binding stoichiometry for Co II :protein and 1:1 binding stoichiometry for Co II :ligand (ligand = fura-2, EGTA or NTA). Ligand dissociation constants at pH 7.0: fura-2 K Co(II) = 8.6 × 10 −9 M (ref. [39] ); EGTA K Co(II) = 7.9 × 10 −9 M (ref. [38] ); NTA K Co(II) = 2.2 × 10 −8 M (ref. [38] ). (NH 4 )Fe(SO 4 ) 2 was titrated into a solution of Tar (16 µM), MgCl 2 (2.7 mM) and GTP (500 µM) in the absence or presence of CobW (50 µM) and UV-visible absorbance recorded at equilibrium to define Fe II speciation (Fe II Tar 2 ε 720 =  19,560 M −1 cm −1 under experimental conditions, Supplementary Fig. 8a ). Data were fit in Dynafit [52] to a model describing 1:1 binding stoichiometry for Fe II :protein and 1:2 binding stoichiometry for Fe II :Tar using β 2,Fe(II) = 4.0 × 10 13 M −2 for Tar at pH 7.0 (ref. [54] ). Experimental data were compared to simulated fits with defined protein K Fe(II) = 10 −6 M, 10 −7 M, allowing limiting K D ≥ 10 −6 M for Mg II GTP-CobW to be determined. Tar stock concentrations were quantified using ε 470 nm = 24,800 M −1 cm −1 (reported value at pH 7.0 (ref. [54] )) and verified by titration with metal stocks (Fe II or Ni II , quantified by ICP-MS). NiSO 4 was titrated into a solution of Tar (20 µM), CobW (10–30 µM), MgCl 2 (2.7 mM) and GTP (100–300 µM) and UV-visible absorbance recorded at equilibrium to determine Ni II speciation (Ni II Tar 2 Δ ε 535 nm = 3.8 (±0.1) × 10 4 M −1 cm −1 relative to ligand only solution; Supplementary Fig. 10a ). Tar stock concentrations were quantified as above. Data were fit using Dynafit [52] to a model describing 1:1 stoichiometry Ni II :protein and 1:2 stoichiometry Ni II :Tar; β 2,Ni(II) = 4.3 (±0.6) × 10 15 M −2 for Tar at pH 7.0 was independently determined by preparing a series of solutions of NiTar 2 ([Ni II ] = 15 µM, [Tar] = 36 µM) with varying EGTA concentrations (0–400 µM) and measuring UV-visible absorbance at equilibrium (following 1–2 h incubation). EGTA K Ni(II) = 5.0 × 10 −10 M at pH 7.0 (ref. [38] ). Data were fit to Eq. ( 5 ) [51] using Kaleidagraph (Synergy Software). [EGTA]_tot/[Ni^II]_tot = 1 - [Ni^IITar_2]/[ Ni^II]_tot + K_D( EGTA)β_2(Tar)( [Tar]_tot/[Ni^IITar_2] - 2)^2[Ni^IITar_2]( 1 - [Ni^IITar_2]/[ Ni^II]_tot)
 (5) CuSO 4 was titrated into a solution of Bca (1.0 mM), CobW (10–30 µM), MgCl 2 (2.7 mM), GTP (100–300 µM) and reductant NH 2 OH (1.0 mM) which quantitatively reduces Cu II to Cu I in the presence of a strong Cu I ligand (e.g. Bca: β 2,Cu(I) = 1.6 × 10 17 M −2 (ref. [38] )). UV-visible absorbance was recorded at equilibrium to define Cu I speciation (Cu I Bca 2 ε 562 = 7900 M −1 cm −1 (ref. [38] )) and data were fit using Dynafit [52] to a model describing 1:1 stoichiometry Cu I :protein and 1:2 stoichiometry Cu I :Bca. ZnCl 2 was titrated into a solution containing quin-2 (10 µM), CobW (10 µM), MgCl 2 (2.7 mM) and GTP (50 µM) and UV-visible absorbance recorded at equilibrium. Quin-2 was quantified using ε 261 nm = 37,000 M −1 cm −1 (ref. [55] ). K Zn(II) for Mg II GTP-CobW was beyond the range of this experiment (significantly tighter than quin-2) and only a limiting affinity was determined ( K Zn(II) < 10 −12 M). Zn II affinity of Mg II GTP-CobW via inter-metal competition Solutions containing CobW (17.9–20.4 µM), MgCl 2 (2.7 mM), GTP (200 µM) and ligand NTA (0.4–4.0 mM) were titrated with CoCl 2 (0.3–3.0 mM) and ZnCl 2 (15.3–25.5 µM) and UV-visible absorbance was recorded at equilibrium to determine Co II occupancy of CobW ( ε 339 nm = 2800 M −1 cm −1 for Co II Mg II GTP-CobW). Details of individual experiments are in Supplementary Table 4 . The total concentration of Co II and Zn II in each solution was limiting, such that both metals were buffered by ligand NTA. Metal speciation was determined from the mass balance relationships given in Eqs. ( 6 – 8 ) (cofactors Mg II GTP omitted for clarity). Thus, K Zn(II) for Mg II GTP-CobW was calculated from the exchange equilibria ( K ex ) in Fig. 4a , relative to known K Co(II) for the protein (Supplementary Table 2 ) and ligand dissociation constants (NTA K Zn(II) = 1.18 × 10 −8 M, K Co(II) = 2.24 × 10 −8 M (ref. [38] )). These calculations are valid given that [M] free ≪ [M] tot (M = Co II or Zn II , buffered by excess NTA), the concentration of non-metalated protein is negligible (Supplementary Fig. 13 ) and potential ternary complexes involving metal, protein and NTA are transient species only with insignificant concentration at thermodynamic equilibrium (varying ratios of buffered metals, [Co II NTA]/[Zn II NTA], were used to confirm consistency of K D values at multiple equilibria; see Fig. 4 and Supplementary Table 4 ). [Co^IINTA] = [Co^II]_tot - [Co^IICobW]
 (6) 
    [Zn^IICobW] = [CobW]_tot - [Co^IICobW]
 (7) 
    [Zn^IINTA] = [Zn^II]_tot - [Zn^IICobW]
 (8) Determination of YeiR and YjiA metal stoichiometries and affinities Investigation of protein–metal interactions and competition experiments to determine metal affinities were performed in 10 mM HEPES pH 7, 100 mM NaCl, 400 mM KCl (chelex treated and N 2 purged) with the inclusion of nucleotides and MgCl 2 as noted in figure legends. Absorbance was recorded using a Lambda 35 UV-visible spectrophotometer (Perkin Elmer). Fluorescence spectra were recorded using a Cary Eclipse fluorescence spectrophotometer (Agilent). Scripts used for data fitting (using Dynafit [52] ) are provided in Supplementary Software 2. CoCl 2 was titrated into a solution of fura-2 ( ε 363 nm = 28,000 M −1 cm −1 , K Co(II) = 8.6 × 10 −9 M (refs. [39] , [53] )) in the presence of YeiR or YjiA and fluorescence emission (510 nm) recorded at equilibrium ( λ ex = 360 nm, 20 °C). Data were fit to a model describing 1:1 Co II :fura-2 and 1:1 Co II :protein binding stoichiometries using Dynafit [52] . NiCl 2 was titrated into a solution of Mf2 ( ε 369 nm = 22,000 M −1 cm −1 , K Ni(II) = 5 × 10 −8 M (refs. [53] , [56] )) in the presence of YeiR or YjiA and the absorbance (323–325 and 365–366 nm) recorded at equilibrium. Data were fit (both wavelengths simultaneously) to a model describing 1:1 Ni II :Mf2 and 1:1 Ni II :protein binding stoichiometries using Dynafit [52] . ZnSO 4 was titrated into a solution of Mf2 ( K Zn(II) = 2 × 10 −8 M (ref. [57] )), PAR ( β 2 Zn(II) = 2 × 10 12 M −2 (ref. [58] )) or quin-2 ( K Zn(II) = 3.7 × 10 −12 M (ref. [55] )) in the presence of YeiR or YjiA and the absorbance (325 and 366 nm Mf2; 500 nm PAR; 265 or 269 nm quin-2) recorded at equilibrium. Concentrations of PAR and quin-2 stocks were determined by direct titration with ZnSO 4 . Data were fit to a model describing 1:1 Zn II :quin-2 and 1:1 Zn II :YjiA binding stoichiometries. Zn:YeiR stoichiometries were fit as 1:1, or allowed to be determined in fitting as described in the text using Dynafit [52] . CuSO 4 was titrated into a solution of Bca (Cu I Bca 2 ε 562 nm = 7900 M −1 cm −1 , β 2 Cu(I) = 10 17.2 M −2 (ref. [59] )) in the presence and absence of YeiR or YjiA (with inclusion of hydroxylamine) and absorbance (562 nm) recorded at equilibrium. Protein Cu I affinity was calculated using Eq. ( 9 ), for the tightest binding event. Calculated affinities were simulated using Dynafit [52] , and overlaid on the data. K_Dβ _2 = ( [P]_tot/[MP]) - 1/( ( [L]_tot/[ML_2] - 2)^2[ML_2])
 (9) (NH 4 )Fe(SO 4 ) 2 was titrated into a solution of Tar (Tar 2 Fe(II) ε 720 nm =  19,000 M −1 cm −1 , β 2 Fe(II) = 10 13.6 M −2 (at pH 7.0) (ref. [54] ) in the presence and absence of YeiR or YjiA and absorbance (720 nm) recorded at equilibrium. Data were fit to a model describing 1:2 Fe II :Tar and 1:1 Fe II :protein binding stoichiometries using Dynafit [52] . MnCl 2 was titrated into a solution of Mf2 ( K Mn(II) = 6.1 × 10 −6 M (ref. [9] )) in the presence of YjiA and the absorbance (330 and 365 nm) recorded at equilibrium. Data were fit (both wavelengths simultaneously) to a model describing 1:1 Mn II :Mf2 and 1:1 Mn II :protein binding stoichiometries using Dynafit [52] . Gel filtration chromatography of YeiR was performed by application of 0.5 mL (10 μM) to a PD-10 Desalting Column prepacked with Sephadex G-25 medium equilibrated with buffer supplemented with 2.7 mM MgCl 2 with or without 20 μM MnCl 2 and eluted with the same buffer. YeiR was incubated with 20 μM MnCl 2 for 20 min prior to application to the column. Protein content of collected fractions was assayed by A 280 nm and Bradford assay, metal content by ICP-MS. Inter-protein competition for Co(II) Experiments were performed in an anaerobic glovebox. YeiR (10 μM) was incubated with GTP (100 μM), MgCl 2 (2.7 mM) and CoCl 2 (8 μM) in 10 mM HEPES pH 7.0, 40 mM NaCl, 160 mM KCl (chelex treated and N 2 purged) for 10 min before addition of CobW (10 μM) (total volume upon CobW addition = 1.1 mL). The mixture was incubated for a further 30 min before application of 1 mL of the incubation reaction to a 1-mL Q anion exchange column (GE Healthcare) equilibrated with 10 mM HEPES pH 7.0, 40 mM NaCl, 160 mM KCl (chelex treated and N 2 purged), collecting the flow through. The column was sequentially eluted with equilibration buffer collecting six 0.5 mL fractions followed by 10 mM HEPES pH 7.0, 200 mM NaCl, 800 mM KCl (chelex treated and N 2 purged) collecting six 0.5-mL fractions. Fractions were analysed for protein content by SDS-PAGE and for metal content by ICP-MS. Controls were conducted concurrently as above but with YeiR or CobW alone. GTPase activity assays CobW (20–50 µM) was incubated with CoCl 2 (0.9 equivalents Co II :protein) and GTP (200 µM) in an anaerobic chamber in N 2 -purged, chelex-treated 10 mM HEPES pH 7.0, 100 mM NaCl, 400 mM KCl. Aliquots of solution taken at various time intervals (0–390 min) were loaded to a 5-mL HiTrap Q HP column (GE Healthcare) equilibrated in buffer (20 mM HEPES pH 7.0, 100 mM NaCl) and eluted with a linear NaCl gradient (100–500 mM NaCl). Nucleotides were detected by UV absorbance (254 nm or 280 nm) and the ratio of GTP:GDP in each sample was calculated by integration of the respective peak areas. Growth of E. coli* strains E. coli* strains used in this work are derived from E. coli MG1655 (DE3) engineered to contain a set of B 12 biosynthesis genes from R. capsulatus [60] , [61] , and Brucella melitensis (B. melitensis) [34] . Strain ED741 ( E. coli* without cobW ) is MG1655 with P lac -T7RNAP-P T7 -cobAIGJFMKLHBROQJD-bluE-C-bluF-PUB-cbiW-VE-P T7 -cobNST while strain ED732 ( E. coli* with cobW ) is MG1655 with P lac - T7 RNAP-P T7 -cobAIGJFMKLHBROQJD-bluE-C-bluF-PUB-cbiW-VE-P T7 -cobWNST. All R. capsulatus and B. melitensis ( cobG, cobR, cobE ) genes were cloned individually in pET3a and subcloned together using the link and lock method [34] . The synthetic operons were transferred into the E. coli genome using CRISPR technology [62] . Although chromosomally integrated B 12 biosynthesis genes are IPTG-inducible under the control of the T7 promoter, in the current experiments IPTG was not added to cell cultures to avoid potential disruptions of cellular metal homoeostasis caused by over-production of metalloproteins. All cultures and media were prepared in plasticware or acid-washed glassware to minimise trace metal contamination. LB medium was inoculated with overnight culture of E. coli* (OD 600 nm = 0.025) and incubated at 37 °C with shaking until OD 600 nm reached ~0.2. Aliquots (5 mL or 50 mL) of this culture were treated with sterile CoCl 2 , H 2 O, EDTA or ZnCl 2 (100× concentrated stocks) to reach final concentrations as specified in figure legends (Figs. 8 b, 9b and Supplementary Figs. 27 , 28a , b, d and 29c ) and incubated under the same conditions for a further 1–4 h. Samples used for RNA extraction were taken 1 h after treatment. Samples for B 12 quantification and OD 600 nm readings were taken 4 h after treatment to ensure detectable corrinoid production. Determination of transcript abundance in E. coli* Aliquots (1 mL) of E. coli* culture from each growth condition were stabilised in RNAProtect Bacteria Reagent (2 mL; Qiagen) and cells pellets were frozen at −80 °C prior to processing. RNA was extracted using an RNeasy Mini Kit (Qiagen) as described by the manufacturer. RNA was quantified by absorbance at 260 nm and treated with DNAse I (2.5 U/μL; Fermentas). cDNA was generated using the ImProm-II Reverse Transcriptase System (Promega) with 300 ng RNA per reaction, and control reactions without reverse transcriptase were conducted in parallel. Transcript abundance was determined using primers 3 and 4 for rcnA , 5 and 6 for zntA , 7 and 8 for znuA , 9 and 10 for rpoD , each pair designed to amplify ~110 bp fragment. Quantitative PCR analysis was carried out in 20 µL reactions using 5 ng of cDNA, 0.8 µM of each appropriate primer and PowerUp SYBR Green Master Mix (Thermo Fisher Scientific). Three technical replicates of each sample (i.e. biological replicate) were analysed using a Rotor-Gene Q 2plex (Qiagen; Rotor-Gene-Q Pure Detection software), plus control reactions without cDNA template for each primer pair. The fold change, relative to the mean of the control condition for each sensor, was calculated using the 2 −ΔΔCT method [63] , with rpoD as the reference gene. C q values were calculated with LinRegPCR after correcting for amplicon efficiency [64] . Intracellular available ∆ G Co(II) under bespoke conditions Intracellular available ∆ G metals were first calculated from available metal concentrations where the cognate sensor is at 1%, 10%, 50%, 90% and 99% of its response (i.e., θ D = 0.01, 0.1, 0.5, 0.9, 0.99; Supplementary Note 1 ). Available metal concentrations corresponding to these fractional occupancies were determined using known metal affinities, DNA affinities, protein abundances and numbers of DNA binding sites determined for Salmonella sensors [9] , using excel spreadsheet (Supplementary Dataset 1 ) and MATLAB code (Supplementary Note 3 ) available in ref. [9] . Fractional responses ( θ D ) of RcnR at bespoke growth conditions were calculated from transcript abundance of rcnA via Eq. ( 10 ): 
    Conditional θ _D = 0.99 - 0.98 ×( fold - change_obs - 1/fold - change_max - 1)
 (10) where fold-change obs is the observed fold-change in rcnA transcript abundance at the bespoke condition and fold-change max is the maximum fold-change in rcnA transcript abundance at the calibration limit (corresponding to maximum abundance); all fold-changes were determined relative to the defined control condition (untreated LB) corresponding to minimum rcnA transcript abundance (see Supplementary Fig. 27c ). Equation ( 10 ) defines maximum and minimum transcript abundances as corresponding to θ D of 0.01 and 0.99, respectively (see Fig. 8a ), and assumes a linear relationship between change in θ D and change in transcript abundance. The intracellular available [Co II ] concentration corresponding to each RcnR θ D was calculated using known metal affinity, DNA affinities, protein abundance, number of DNA binding sites determined for Salmonella RcnR [9] , to calculate the Co II -dependent response of E. coli RcnR (93% sequence identity) using excel spreadsheet (Supplementary Dataset 1 ) and MATLAB code (Supplementary Note 3 ) available in ref. [9] . The intracellular available Δ G Co(II) for each condition was calculated using Eq. ( 11 ), where [Co II ] is the intracellular available Co II concentration, R (gas constant) = 8.314 × 10 −3 kJ K −1 mol −1 and T (temperature) = 298.15 K (see Supplementary Note 1 ). Intracellular available ΔG_Co(II) = RTln[ Co^II]
 (11) E stimation of intracellular available ∆ G Zn(II) in LB media Fractional responses ( θ D ) of Zur and ZntR in LB media were calculated from transcript abundance of znuA and zntA , via Eqs. ( 10 ) and ( 12 ), respectively: 
    Conditional θ _D = 0.01 + 0.98 ×( fold - change_obs - 1/fold - change_max - 1)
 (12) where fold-change obs is the observed fold-change in transcript abundance in LB and fold-change max is the maximum fold-change in transcript abundance at the calibration limit (corresponding to maximum abundance); all fold-changes were determined relative to defined control conditions corresponding to minimum transcript abundance (see Supplementary Fig 28a, b ). Equation ( 12 ) defines maximum and minimum transcript abundances as corresponding to θ D of 0.99 and 0.01, respectively, and assumes a linear relationship between change in θ D and change in transcript abundance. The intracellular available [Zn II ] concentration corresponding to each θ D was calculated using known metal affinities, DNA affinities, protein abundance, number of DNA binding sites determined for Salmonella homologues, to calculate the Zn II -dependent responses of E. coli ZntR and Zur (both >92% sequence identity to Salmonella ) using excel spreadsheet (Supplementary Dataset 1 ) and MATLAB code (Supplementary Note 3 ) available in ref. [9] . The intracellular available Δ G Zn(II) was calculated using Eq. ( 13 ), where [Zn II ] is the intracellular available Zn II concentration, R (gas constant) = 8.314 × 10 −3 kJ K −1 mol −1 and T (temperature) = 298.15 K (see Supplementary Note 1 ). Intracellular available ΔG_Zn(II) = RTln[ Zn^II]
 (13) Quantification of vitamin B 12 in E. coli* cultures Aliquots (20 mL) of E. coli* culture from each growth condition were taken, and cell pellets frozen at −20 °C. To quantify corrin production (assumed to be predominantly B 12 , since E. coli* contains genes for the complete pathway), E. coli* pellets were thawed, resuspended in H 2 O (0.2 mL), boiled for 15 min (95 °C) and centrifuged to remove cell debris. An aliquot (10 µL) of each supernatant was applied to Salmonella typhimurium AR2680 ( ΔmetE, ΔcbiB ) pre-innoculated bioassay plates [65] , and incubated at 37 °C overnight. Plates were imaged together with a 1-cm 2 reference area on black background (see example in Supplementary Data 2 ) using a Gel-Doc XR + gel documentation system (BioRad; ImageLab software). Images were analysed in MATLAB using the code in Supplementary Software 1 to determine the growth area (in cm 2 ) of each sample. A calibration curve relating growth areas to B 12 concentration was generated using B 12 standards (cyanocobalamin; 1–100 nM; quantified by A 360 nm = 27,500 M −1 cm −1 at pH 10 (ref. [66] )) in parallel with E. coli* lysates, using the same batch of bioassay plates (Supplementary Fig. 29a, b ). To determine the number of cells in each sample, solutions of E. coli* at varying cell densities (OD 600 nm = 0.2–0.9) were prepared, serially diluted (2000-fold), and the number of cells per mL quantified using a CASY® cell counter. The resulting correlation factor (4.4 ± 0.1 × 10 8 cells mL −1 OD 600 nm −1 ) was used to convert OD 600 nm to cell number (Supplementary Fig. 29c, d ). Metal content of E. coli* cells Aliquots (20 mL) of E. coli* culture from each growth condition were taken and pellets were washed twice with 0.5 M sorbitol, 200 μM EDTA, 20 mM Tris pH 8.5. Cell pellets were suspended in ultrapure 65% (v/v) HNO 3 (0.4 mL) to digest (>24 h), then diluted tenfold in 2.5% HNO 3 before metal analysis by ICP-MS. Statistics and reproducibility Sample sizes were chosen based on prior experimental experience, and to give consistent results, following convention in the literature for equivalent analyses. Experiments designed to derive quantitative values used to model or test calculations of metalation were performed in triplicate or more ( n = 3–5) to enable calculation of SD (listed in Tables or shown as error bars in figures). The number of independent experiments or biologically independent samples is shown in figure legends or footnotes of Tables. Reporting summary Further information on research design is available in the Nature Research Reporting Summary linked to this article.